Real-timein vivoimaging of the beating mouse heart at microscopic resolution Real-time imaging of moving organs and tissues at microscopic resolutions represents a major challenge in studying the complex biology of live animals. Here we present a technique based on a novel stabilizer setup combined with a gating acquisition algorithm for the imaging of a beating murine heart at the single-cell level. The method allows serial in vivo fluorescence imaging of the beating heart in live mice in both confocal and nonlinear modes over the course of several hours. We demonstrate the utility of this technique for in vivo optical sectioning and dual-channel time-lapse fluorescence imaging of cardiac ischaemia. The generic method could be adapted to other moving organs and thus broadly facilitate in vivo microscopic investigations. Intravital microscopy, computational advances in optical imaging and the development of novel molecular probes (new biological reporters [1] and more efficient fluorochromes [2] ) have each contributed to significant advances in in vivo biology. One of the major advantages of optical microscopy over other imaging modalities is its high spatio-temporal resolution [3] , [4] . Imaging, however, is often still done in optically transparent tissues and model systems (such as embryos or fish) or on isolated organ models (for example, perfused heart preparations). Imaging can also involve exteriorization and immobilization of entire organs on pedicles (for example, exteriorized liver) or the use of dorsal skin window chambers [5] . These methods are not always faithful or practical, and are not commonly compatible with long-term serial observations and survival. Furthermore, measurements are often profoundly affected by respiratory and cardiac motion. Thus, motion compensation and tissue stabilization are two major practical challenges currently faced by researchers using intravital microscopy in murine models [6] . To overcome these issues, a number of different approaches [7] , [8] , [9] , [10] , [11] , [12] , [13] , [14] have been proposed, including the use of restraining cover slips ( Supplementary Fig. S1 ) or suctioning devices. Although reducing motion to some degree, these approaches are far from perfect, and often induce tissue damage or alter physiology. Here, we present a new approach for real-time microscopic imaging, which involves a combination of motion stabilization and an algorithm for image acquisition during advanced cardiopulmonary gating. We use this approach for in vivo confocal and multiphoton microscopy imaging of the beating murine heart at (sub)cellular resolution. This method not only enables prolonged observation for periods up to several hours but also allows repeated imaging over several days, making it particularly suitable for studies of inflammatory responses that play out over several days rather than minutes to hours. Finally, we demonstrate that the described technique is capable of both optical sectioning in confocal and multiphoton mode as well as time-lapse fluorescence imaging allowing individual cells to be tracked in the beating mouse heart. The method is simple and induces no measurable physiological damage as the imaging objective is not in direct contact with the tissue being imaged. Description of the imaging setup The image stabilization approach consists of two distinct and integrated strategies. First, we designed and implemented a specialized tissue motion stabilizer ( Fig. 1 ; Supplementary Fig. S2 ), which reduces artifacts induced by respiratory and cardiac motion ( Fig. 2 ); such motion is typically in the order of several millimetres. Second, we used a real-time processing approach ( Fig. 3a ) to trigger stabilized image extraction at appropriate phases of the respiratory and cardiac cycles using a retrospective electrocardiogram (ECG)-gating technique [15] . The custom-designed stabilizer ( Fig. 1 ; Supplementary Fig. S2 ) consists of a 3-cm-long rigid metal shaft and a flat ring at one end ( Fig. 1b,c ). The ring is bonded to the myocardium and thereby provides a contact-free central area in which a water-immersion objective rests over unaltered myocardium. Bonding to the myocardium is achieved by coating the underside of the ring with a thin layer of ~50 μm of Dermabond, a clinical grade bonding agent that is FDA approved for human surgical use and commonly used in cardiac surgery. The ring is then gently placed on the area of the heart to be imaged and is in direct contact with the visceral (that is, inner layer) of the epicardium. Thereafter, the heart is returned to its original position ( Fig. 1d,e ). The only pressure remaining is the one induced by the heart itself while contracting against the stabilizer ring, similar as the heart beating against the chest wall. For this study, the ring was maintained at an incline of 30°, but this angle can be adjusted for other regions of the heart as necessary. The other end of the stabilizer was mounted on a monolithic tristage base plate to allow 6 degrees of freedom. 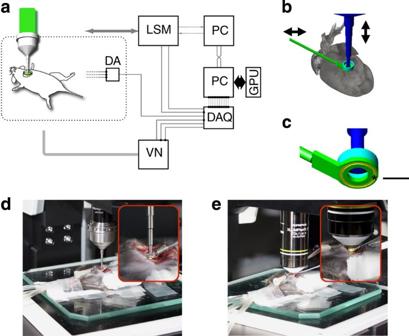Figure 1: Experimental setup and stabilizer design. (a) Experimental setup. DA, differential amplifier; DAQ, data acquisition card; GPU, graphic processing unit; LSM, laser scanning microscope; VN, ventilator. The DAQ card controls all triggers, measures microscope timing, and records both ECG and lung airway pressure. (b) Three-dimensional schematic model of the motion compensation stabilizer. The underside of the ring's stabilizer was bonded to the surface of the heart. The position of the stabilizer could be adjusted in both the horizontal and vertical planes via a monolithic tristage base plate. The stabilizer robustly suppressed artifacts caused by respiration and cardiac contractions (Fig. 2;Supplementary Fig. S1). The stabilizer was filled with a saline solution to provide index matching for the imaging objectives and to prevent the underlying myocardium from drying out. (c) Bottom view of the stabilizer. A shallow groove (yellow ring) was carved out in the bottom part of the stabilizer to increase the contact area between the stabilizer and the bonding material, and thus ensure better attachment to the heart. Scale bar, 2 mm. (d,e) Pictures of the stabilizing setup during live imaging of the heart using either (d) a stick objective (×20 IV-OB13F20W20; Olympus) or (e) a water-immersion objective (×20 XLUMPLANFL; Olympus). Figure 1: Experimental setup and stabilizer design. ( a ) Experimental setup. DA, differential amplifier; DAQ, data acquisition card; GPU, graphic processing unit; LSM, laser scanning microscope; VN, ventilator. The DAQ card controls all triggers, measures microscope timing, and records both ECG and lung airway pressure. ( b ) Three-dimensional schematic model of the motion compensation stabilizer. The underside of the ring's stabilizer was bonded to the surface of the heart. The position of the stabilizer could be adjusted in both the horizontal and vertical planes via a monolithic tristage base plate. The stabilizer robustly suppressed artifacts caused by respiration and cardiac contractions ( Fig. 2 ; Supplementary Fig. S1 ). The stabilizer was filled with a saline solution to provide index matching for the imaging objectives and to prevent the underlying myocardium from drying out. ( c ) Bottom view of the stabilizer. A shallow groove (yellow ring) was carved out in the bottom part of the stabilizer to increase the contact area between the stabilizer and the bonding material, and thus ensure better attachment to the heart. Scale bar, 2 mm. ( d , e ) Pictures of the stabilizing setup during live imaging of the heart using either ( d ) a stick objective (×20 IV-OB13F20W20; Olympus) or ( e ) a water-immersion objective (×20 XLUMPLANFL; Olympus). 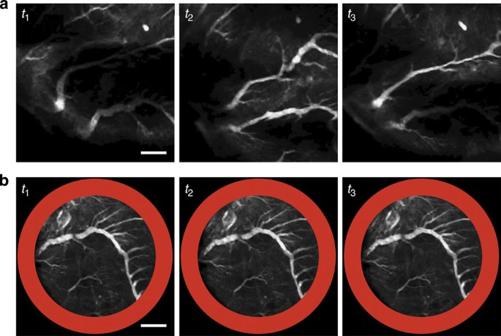Figure 2: Holder stabilization. Whole-field view of a beating heart (a) in the absence, or (b) in the presence of the motion compensation stabilizer. Fluorescent signals shown are from Angiosense-680 (Ex 680 nm and Em 700 nm), a vascular pool imaging agent, which was injected intravenously 5 min before imaging. In both cases (a,b), frames were acquired consecutively at timet1,t2,t3and at a constant speed. The red ring represents the profile of the motion compensation stabilizer. As seen clearly in (a), lack of stabilization rendered images useless owing to the enormous range of motion (several millimetres). Images were acquired using a ×2 objective (XL Fluor 2×/340 NA 0.14). Scale bars, 500 μm. Full size image Figure 2: Holder stabilization. Whole-field view of a beating heart ( a ) in the absence, or ( b ) in the presence of the motion compensation stabilizer. Fluorescent signals shown are from Angiosense-680 (Ex 680 nm and Em 700 nm), a vascular pool imaging agent, which was injected intravenously 5 min before imaging. In both cases ( a , b ), frames were acquired consecutively at time t 1 , t 2 , t 3 and at a constant speed. The red ring represents the profile of the motion compensation stabilizer. As seen clearly in ( a ), lack of stabilization rendered images useless owing to the enormous range of motion (several millimetres). Images were acquired using a ×2 objective (XL Fluor 2×/340 NA 0.14). Scale bars, 500 μm. 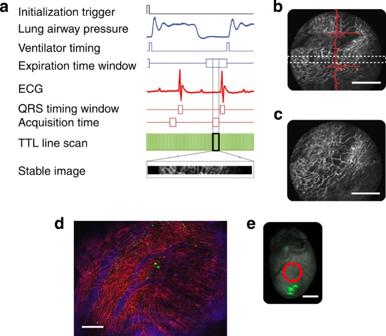Figure 3: Image reconstruction principle and data processing. (a) Timing diagram used for the gated acquisition of images. From top to bottom: TTL initialization trigger, lung airway pressure, TTL ventilator timing, acquisition time window at the end of the expiration, ECG, timing window showing the QRS complex, end-diastolic acquisition time with minimal left ventricular motion, TTL line scan data obtained from the microscope (relative to the image acquired), a section of the image from within the timing window corresponding to a specific portion of the ECG cycle as well as to a well-defined phase of the respiratory cycle. (b) Raw image acquired. Motion artifacts are still visible and their effects vary in accordance to the different phases of the ECG cycle (red line). Using a retrospective ECG-gating technique on each acquired image, only data that fell within the two white dotted lines and corresponded with the time-gating window in (a) were considered. Scale bar, 200 μm. (c) The acquisition of multiple consecutive images leads to a varied collection of sampled regions. Scale bar, 200 μm. (d) Reconstructed image of the beating heart. Red represents the fluorescence lectin signal from stained capillaries; blue represents the fluorescence signal produced by the blood pool imaging agent Angiosense-680; and green represents the GFP-expressing cells. The heart sustained an ischaemia reperfusion injury (for 30 min) before being injected with GFP-expressing cells in the apex. Imaging was performed 24 h post injury; the image shows migrating cells in the inflamed zone. Scale bar, 200 μm. (e) Fluorescence reflectance image of the heart shown in (d). Green represents the fluorescence signal of the GFP-expressing cells injected into the heart's apex. The red circle indicates the effective area where the stabilizer was positioned. All images were taken with the stabilizer placed on equivalent areas. Scale bar, 2 mm. Images for (d) were acquired using a ×10 air objective (Olympus, UPlanFL N NA 0.30), and for (b,c) using a ×6 MicroProbe objective (Olympus, IV-OB13F20W20). Full size image Figure 3: Image reconstruction principle and data processing. ( a ) Timing diagram used for the gated acquisition of images. From top to bottom: TTL initialization trigger, lung airway pressure, TTL ventilator timing, acquisition time window at the end of the expiration, ECG, timing window showing the QRS complex, end-diastolic acquisition time with minimal left ventricular motion, TTL line scan data obtained from the microscope (relative to the image acquired), a section of the image from within the timing window corresponding to a specific portion of the ECG cycle as well as to a well-defined phase of the respiratory cycle. ( b ) Raw image acquired. Motion artifacts are still visible and their effects vary in accordance to the different phases of the ECG cycle (red line). Using a retrospective ECG-gating technique on each acquired image, only data that fell within the two white dotted lines and corresponded with the time-gating window in ( a ) were considered. Scale bar, 200 μm. ( c ) The acquisition of multiple consecutive images leads to a varied collection of sampled regions. Scale bar, 200 μm. ( d ) Reconstructed image of the beating heart. Red represents the fluorescence lectin signal from stained capillaries; blue represents the fluorescence signal produced by the blood pool imaging agent Angiosense-680; and green represents the GFP-expressing cells. The heart sustained an ischaemia reperfusion injury (for 30 min) before being injected with GFP-expressing cells in the apex. Imaging was performed 24 h post injury; the image shows migrating cells in the inflamed zone. Scale bar, 200 μm. ( e ) Fluorescence reflectance image of the heart shown in ( d ). Green represents the fluorescence signal of the GFP-expressing cells injected into the heart's apex. The red circle indicates the effective area where the stabilizer was positioned. All images were taken with the stabilizer placed on equivalent areas. Scale bar, 2 mm. Images for ( d ) were acquired using a ×10 air objective (Olympus, UPlanFL N NA 0.30), and for ( b , c ) using a ×6 MicroProbe objective (Olympus, IV-OB13F20W20). Full size image The use of this stabilizer setup resulted in near complete suppression of respiratory and cardiac motion artifacts ( Figs 2 and 3b ). During the entire acquisition period, the stabilizer ring was kept filled with physiological saline solution ( Supplementary Fig. S2 ) to provide index matching for the imaging objective and prevent tissue from drying out. To access the heart without altering the position of the ring, we used minimally invasive water-immersion MicroProbe objectives (Olympus). Owing to their small diameters (1.3 mm) and working distances (200 μm), these objectives could be easily accommodated within the ring ( Fig. 1d ; Supplementary Fig. S2 ). Likewise, they also provided the capability for deep (100 μm) tissue imaging. To image deeper tissue structures, we utilized multiphoton imaging ( Supplementary Fig. S3 ) in combination with a large working distance (2 mm) water-immersion objective ( Fig. 1e ). For this, the top side of the ring was machined so as to accommodate a seal-proof 1-mm-tall plastic ring extension. A layer of 200 μm to 2 mm of water was present between the heart and the imaging lens, and there was thus no contact between the tissue and the objective ( Fig. 1e ; Supplementary Fig. S2 ). The objective and the ring are thus two distinct units that are not connected to each other. In addition, a shallow groove ( Fig. 1c ) was carved out of the underside of the ring to increase the contact area between the glue and the surface of the stabilizer, and thus maximize the bond between the stabilizer and the heart. Finally, to maintain both the ring and its enclosed physiological solution at 37 °C, both the objective and the stabilizer were thermally controlled via resistive heaters and thermistors. Retrospective gating acquisition and real-time processing While the mechanical approach was relatively efficient at reducing the heart's range of motion by several orders of magnitude ( Fig. 2 ), residual motion artifacts were still present in the acquired images ( Fig. 3b ); this is presumably a result of the cardiac contractions during the microscope acquisition time (approximately one beat occurs every 200 ms during deep anaesthesia in mice). This problem was particularly troublesome during high-resolution imaging, where the acquisition time is comparable to, or longer than, one ECG cycle ( Fig. 2a ). To overcome this issue, we implemented both cardiac and respiratory gating. As animals were mechanically ventilated in a pressure-cycle mode, image acquisition extraction could be gated to a particular phase of the respiratory cycle synchronized with the cardiac cycle (see timing diagram in Fig. 3a ). Specifically, we chose a ventilator timing window of 90 ms near the end of expiration that was achieved with a constant delay occurring immediately after the initial ventilation trigger. For the cardiac cycle, we chose an image acquisition timing window of 15 ms following the appearance of the P wave and coinciding with end diastole in the ventricle ( Fig. 3a ; Supplementary Fig. S4 ). When only cardiac gating was used, respiratory artifacts strongly affected the reconstructions ( Supplementary Fig. S5 ). As a result, this strategy was abandoned. Multiple-gated images within the same phase of the respiratory and cardiac cycles were then consecutively acquired (white box, Fig. 3b ). These gated data were then fused to generate a final reconstructed image ( Fig. 3c ), which was built in real time during acquisition. Analogously, a prospective gating approach could be adopted in a similar fashion using microscopy systems that allow fast triggering of image scanning. Imaging cardiac tissue in vivo We subsequently tested the in vivo stabilization method in a mouse model of ischaemia reperfusion injury, in which we tracked the migration of exogenously administered cells ( Fig. 3d ). We chose this model because it is a commonly used and clinically relevant injury model [16] , and because it allows visualization of leucocyte entry into the ischaemic tissue. The left anterior descending artery was temporarily occluded for 30 min to induce the ischaemic injury and to trigger an inflammatory response. Green fluorescent protein (GFP)-expressing cells, freshly isolated from the bone marrow of donor mice, were subsequently injected into the cardiac apex ( Fig. 3e ), and live mice were imaged 24 h later. Once the stabilizer was in place (red ring in Fig. 3e ), Griffonia simplicifolia-I lectin [17] was injected intravenously, which selectively stains mouse endothelial cells. Angiosense-680, an in vivo blood pool imaging agent, was also injected to visualize vascular perfusion. In the reconstructed image ( Fig. 3d ; Supplementary Fig. S6 ), GFP-expressing cells are clearly visible in an area distant from the injection site, a finding that suggests cell migration. During a typical imaging session, we monitored multiple physiological parameters (heart rate, respiratory rate, temperature, blood pressure, oxygenation, hydration, and so on). In addition, to determine whether the stabilizer had any effect on tissue perfusion, we imaged both lectin and Angiosense-680 in real time ( Fig. 4 ; Supplementary Fig. S7 ). We were able to demonstrate that capillary perfusion was normal ( Fig. 4 ; Supplementary Movie 1 ). ECG data before, during and after intravital imaging sessions showed normal cardiac electrical activity ( Supplementary Fig. S8 ). In addition, heart function was not impaired during or after the imaging sessions. Using cardiac magnetic resonance imaging, we quantified the left ventricular ejection fraction ( n =4 mice) 2 days after intravital imaging, comparing it with the ejection fraction obtained before the imaging sessions. Ventricular ejection fractions were similar to pre- and post-intravital imaging ( Supplementary Fig. S9 ). Moreover, CD11b immunohistochemistry staining of heart tissue following intravital imaging showed no inflammatory activity as a result of intravital imaging ( Supplementary Fig. S10 ). Finally, use of fluorescent microspheres, the gold standard method to measure organ perfusion in a non-survival experiment, did not demonstrate any micro-perfusion abnormalities in the imaging area as compared with control myocardium ( Supplementary Fig. S11 ). 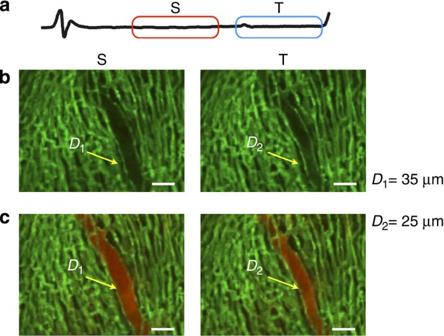Figure 4: Vasculature perfusion. Time-lapse fluorescence imaging of heart perfusion using a vascular pool imaging agent injected via tail vain as inSupplementary Fig. S9. (a) Frames S and T are taken at two different time-gating windows within the ECG. Images taken before (b) and after (c) perfusion. Changes in the vessel diameter are evident for the two phases. Fluorescent lectin staining of capillaries is depicted in green; fluorescent signal from the vascular pool agent Angiosense-680 is depicted in red. Scale bars, 50 μm. Figure 4: Vasculature perfusion. Time-lapse fluorescence imaging of heart perfusion using a vascular pool imaging agent injected via tail vain as in Supplementary Fig. S9 . ( a ) Frames S and T are taken at two different time-gating windows within the ECG. Images taken before ( b ) and after ( c ) perfusion. Changes in the vessel diameter are evident for the two phases. Fluorescent lectin staining of capillaries is depicted in green; fluorescent signal from the vascular pool agent Angiosense-680 is depicted in red. Scale bars, 50 μm. Full size image Characterization of the imaging resolution Our next aim was to determine the extent of residual motion after placement of the stabilizer on the cardiac surface. For this, we injected fluorescein isothiocyanate-labelled fluorescent beads (diameter of 5 μm) directly in the left ventricle ( Fig. 5a ). After a few minutes, a small percentage of the beads became trapped in the myocardial microvessels, and thus served as reliable fiducial markers. 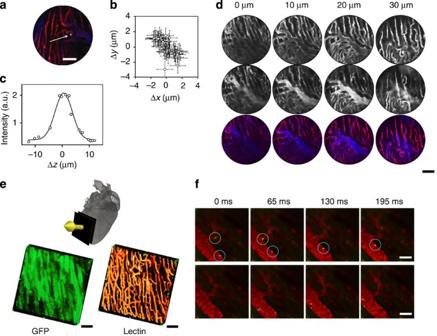Figure 5:In vivoresolution and heart imaging. (a) A stabilized image of a fluorescein isothiocyanate (FITC)-labelled bead (diameter: 5 μm), trapped within a microvessel, used to determine the overall stabilized imaging resolution. Red: lectin-stained capillaries; blue: Angiosense-680 (blood pool imaging agent); yellow: the FITC-labelled bead. Scale bar, 50 μm. (b) The planar position coordinates of the trapped bead are plotted at different time points to allow acquisition of consecutive unprocessed images. Error bars (+/−1 μm) correspond to the error in the position determination of the centroid in the acquired image. A resolution of 4 μm was achieved with hardware stabilization. Gating improved the resolution to 2 μm. Under suboptimal positioning of the stabilizer owing to the presence of dishomogeneities in the bonding agent layer, or when the holder is poorly aligned with the heart's surface, a reduced resolution of 4 μm along thexdirection and 11 μm along theydirection was obtained (Supplementary Movie 1) (c) Characterization of the axial resolution achieved using the gating modality in combination with the motion compensation stabilizer. Here, the axial position of the bead within the imaging time-gating window (defined inFig. 1) was determined at different depths. (d)In vivooptical sectioning of the myocardium. Top row, lectin; mid row, Angiosense-680; bottom row, fusion of top and mid row images. Images were taken at different depths in 10-μm increments, using a ×20 MicroProbe objective. Scale bar, 50 μm. (e) Optical sectioning along the indicated direction (yellow arrow) allowed three-dimensional reconstructions in a GFP-expressing mouse. Green: GFP-expressing myocytes; orange: lectin. Scale bars, 50 μm. (f) Time-lapse (65 ms step) fluorescence imaging allowed tracking of cellsin vivoin the beating heart (green: Rhodamine 6G-stained leucocytes; red: vessels stained with Angiosense-680). Top row, the blue circle highlights a leucocyte rolling along the inner surface of the vessel, whereas the leucocyte in the green circle is in the lumen of the vessel and is therefore travelling faster. Bottom row shows a leucocyte initiating rolling. Shadows within the vessels represent red blood cells (also seeSupplementary Movies 2and3). Scale bars, 20 μm. Figure 5b shows the planar position coordinates of a single bead plotted at different time points during consecutively acquired images. Our findings indicated that hardware stabilization results in a planar resolution of 4 μm. This resolution, which can be greatly improved using the above-described gated acquisition approach, is primarily determined by two factors. Aside from obvious considerations regarding the optical components of the setup, the first factor is the reliability with which we can capture the beating heart at the same time point in the respiratory and heart cycles. The second determining factor is the reproducibility of this time point over multiple image acquisitions. Using the above-described gating, we were able to obtain a planar resolution of ~2 μm for a stabilized image. Figure 5: In vivo resolution and heart imaging. ( a ) A stabilized image of a fluorescein isothiocyanate (FITC)-labelled bead (diameter: 5 μm), trapped within a microvessel, used to determine the overall stabilized imaging resolution. Red: lectin-stained capillaries; blue: Angiosense-680 (blood pool imaging agent); yellow: the FITC-labelled bead. Scale bar, 50 μm. ( b ) The planar position coordinates of the trapped bead are plotted at different time points to allow acquisition of consecutive unprocessed images. Error bars (+/−1 μm) correspond to the error in the position determination of the centroid in the acquired image. A resolution of 4 μm was achieved with hardware stabilization. Gating improved the resolution to 2 μm. Under suboptimal positioning of the stabilizer owing to the presence of dishomogeneities in the bonding agent layer, or when the holder is poorly aligned with the heart's surface, a reduced resolution of 4 μm along the x direction and 11 μm along the y direction was obtained ( Supplementary Movie 1 ) ( c ) Characterization of the axial resolution achieved using the gating modality in combination with the motion compensation stabilizer. Here, the axial position of the bead within the imaging time-gating window (defined in Fig. 1 ) was determined at different depths. ( d ) In vivo optical sectioning of the myocardium. Top row, lectin; mid row, Angiosense-680; bottom row, fusion of top and mid row images. Images were taken at different depths in 10-μm increments, using a ×20 MicroProbe objective. Scale bar, 50 μm. ( e ) Optical sectioning along the indicated direction (yellow arrow) allowed three-dimensional reconstructions in a GFP-expressing mouse. Green: GFP-expressing myocytes; orange: lectin. Scale bars, 50 μm. ( f ) Time-lapse (65 ms step) fluorescence imaging allowed tracking of cells in vivo in the beating heart (green: Rhodamine 6G-stained leucocytes; red: vessels stained with Angiosense-680). Top row, the blue circle highlights a leucocyte rolling along the inner surface of the vessel, whereas the leucocyte in the green circle is in the lumen of the vessel and is therefore travelling faster. Bottom row shows a leucocyte initiating rolling. Shadows within the vessels represent red blood cells (also see Supplementary Movies 2 and 3 ). Scale bars, 20 μm. Full size image To measure the axial image resolution, mice were positioned on a translation stage, which provided motion along the vertical axis with nanometre accuracy. Measurements were obtained along the z axis by moving the mouse (and therefore the heart) along the vertical direction. Both the mouse and the ring holder were located on the same moving plate while three-dimensional stacks were acquired. The axial resolution of the current setup was determined as 7 μm by measuring the axial position of a bead at different depths within the heart, as well as within the imaging time-gating window ( Fig. 5c ), as defined in Fig. 3a . A trade-off exists between imaging speed, resolution and acquisition time for the two imaging approaches ( Table 1 ). In essence, each parameter can be adjusted to enable optimal imaging of different biological tissues. For example, to obtain high signal-to-noise ratio images, using the gated mode (pro- or retrospectively), at low acquisition rates (<5 frames per second) is more appropriate. By contrast, when imaging fast dynamic events such as leucocytes moving within vessels, a free running mode with an acquisition rate of 15 frames per second is preferable. Table 1 Comparison of imaging resolution for different stabilization techniques. Full size table Furthermore, we also compared our stabilized reconstructed images with postmortem images acquired in the same position ( Supplementary Fig. S12 ). This not only verified a good correlation between the two image sets, but also demonstrated the robustness of the technique. Thus, the image stabilizer, when used in combination with gated acquisition, provides superior motion compensation, which in turn facilitates high-resolution imaging. The view-sharing approach adopted here may be new for high-resolution intravital microscopic imaging but is well established for cardiac magnetic resonance imaging [18] . We subsequently applied this methodology to in vivo optical sectioning of the beating heart. This was done by moving the imaging objective along the vertical axis so as to obtain gated reconstructed images at different depths within the myocardium. Stabilized images obtained at four different depths are shown in Fig. 5d . Here, fluorescent contrast was obtained using lectin and Angiosense-680 perfusion. If more detailed microvascular analysis is required, three-dimensional renderings of the beating heart could be obtained (as illustrated in Fig. 5e ) by increasing the number of planes up to the time-gated axial resolution limit. Imaging leucocyte recruitment Given that the tissue stabilizer enables such a high degree of motion, we also used it for video rate imaging. This application is particularly useful for studying leucocyte recruitment in real time. To the best of our knowledge, this is the first time that leucocytes have been successfully imaged in the beating heart. After ischaemia reperfusion injury, we found that Rhodamine 6G-labelled leucocytes could easily be identified within the vessel. Indeed, individual leucocytes could be clearly seen rolling along the endothelium ( Fig. 5f ). In Fig. 5f , we show four consecutive frames obtained at a speed of 15 frames per second. Thus, fluorescence time-lapse acquisitions of the stabilized heart ( Supplementary Movies 2 and 3 ), coupled with real-time processing of cell and vessel segmentation, enabled individual leucocytes to be tracked and counted in the beating heart. As a result, this technique opens up interesting possibilities for in vivo flow cytometry of the heart ( Fig. 6 ). 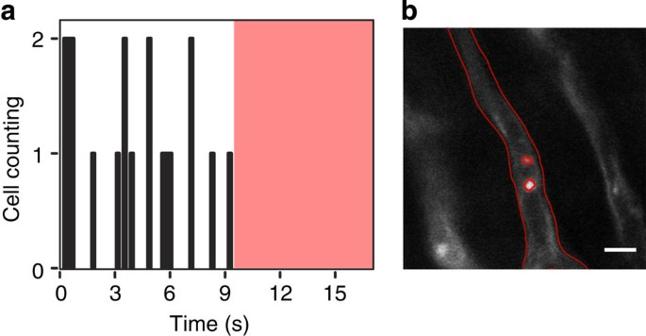Figure 6:In vivoflow cytometry in the beating heart. (a) Number of leucocytes passing through the imaged capillary as a function of time. Images were acquired at 15 frames per second. The red shaded area indicates the time during which no leucocytes were transiting the vessel (Supplementary Movies 2and3). (b) An image of the region of interest, where cells were counted. Segmentation was performed to delineate the border of the vessel and the leucocytes. Leucocytes were stained with Rhodamine 6G (Ex 520 nm and Em 550 nm), injected via tail vein. Capillaries were stained with lectin. Images were acquired using a ×25 water-immersion objective (Olympus, XLPlan N NA 1.05). Scale bar, 10 μm. Figure 6: In vivo flow cytometry in the beating heart. ( a ) Number of leucocytes passing through the imaged capillary as a function of time. Images were acquired at 15 frames per second. The red shaded area indicates the time during which no leucocytes were transiting the vessel ( Supplementary Movies 2 and 3 ). ( b ) An image of the region of interest, where cells were counted. Segmentation was performed to delineate the border of the vessel and the leucocytes. Leucocytes were stained with Rhodamine 6G (Ex 520 nm and Em 550 nm), injected via tail vein. Capillaries were stained with lectin. Images were acquired using a ×25 water-immersion objective (Olympus, XLPlan N NA 1.05). Scale bar, 10 μm. Full size image Imaging myocytes at subcellular resolution Finally, the technique is capable of high-resolution imaging of individual cells. Arguably, the next frontier in in vivo imaging is the ability to improve spatial resolution approximating that of cellular in vitro imaging. Here, we used Hoechst 33258 for topical staining of individual myocyte nuclei ( Fig. 7 ). As clearly seen in these images, even intranuclear structures (nucleoli) can be resolved in the beating heart. 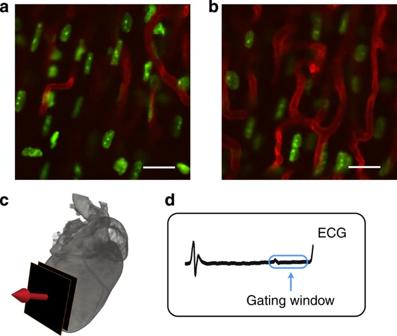Figure 7: High-resolution imaging of myocytes in the beating heart. (a,b) Stabilized fluorescence images of myocyte nuclei obtained at two different depths within the beating heart. Both subcellular and subnuclear structures are clearly resolved. Green: fluorescent Hoechst 33258 staining of myocytes; red: fluorescent lectin staining of capillaries. Scale bar, 20 μm. (c) The red arrow indicates the imaging direction. (d) ECG trace showing the image acquisition time window (blue box). Figure 7: High-resolution imaging of myocytes in the beating heart. ( a , b ) Stabilized fluorescence images of myocyte nuclei obtained at two different depths within the beating heart. Both subcellular and subnuclear structures are clearly resolved. Green: fluorescent Hoechst 33258 staining of myocytes; red: fluorescent lectin staining of capillaries. Scale bar, 20 μm. ( c ) The red arrow indicates the imaging direction. ( d ) ECG trace showing the image acquisition time window (blue box). Full size image We have established a new technique for motion compensation in rapidly moving tissue using a combination of mechanical stabilization and cardiorespiratory-gated acquisitions. We demonstrated in vivo microscopy imaging, in both confocal and multiphoton mode, in the beating mouse heart for up to 4 h over several days. No discernible tissue damage, inflammation or perturbation of cardiac function was observed during or following imaging sessions. The technique was also shown to be capable of tracking cell migration in vivo . Dual-channel fluorescence time-lapse imaging not only enabled the counting of passing leucocytes via in vivo flow cytometry (seconds), but also allowed the visualization of both microvascular rolling and extravasation of leucocytes into injured myocardium (minutes) as well as slower tissue migration within the myocardium over prolonged periods (hours). Moreover, we were able to obtain true four-dimensional information (the fourth dimension being time) in the beating heart. Physiological motion is arguably the most significant obstacle preventing reliable in vivo imaging (aside from light penetration and scattering in optically opaque tissues). To overcome motion, a number of alternative approaches [7] , [8] , [9] , [10] , [11] , [12] , [13] , [14] have been proposed, including the use of restraining cover slips or suctioning devices. While reducing motion to some degree, these approaches, however, are far from perfect. They rarely allow complete immobilization of tissue, are often not compatible with long (hours) imaging sessions and can also damage or alter the tissue of interest. These problems are exacerbated in the beating heart, which has considerable (mm) excursions in multiple dimensions. For example, the mechanical pressure induced by a compressive cover slip often causes severe strain on the organ, while insufficient restraint results in artifacts and lack of reproducibility in motion ( Supplementary Fig. S1 ). Recently, suctioning devices have been shown to be a useful adjunct for lung imaging [7] . However, the lung is not as mechanical rigid and stiff as the heart. We thus found that while suctioning devices were effective in reducing motion artifacts in the heart, they unfortunately caused severe damage to the myocardium over prolonged imaging sessions, owing to the high negative pressure required to achieve appropriate immobilization. Another approach to 'freezing' moving objects is by ultrafast imaging. Bright field microscopy combined with fast CCD acquisition is indicated only for optically transparent tissues and models systems while offering poor axial resolution and extremely low signal-to-noise ratio in adult mice hearts. Recently developed ultrafast multipoint scanning imaging techniques such as spinning disk microscopy or confocal linescan CCD microscopy offer high frame rate acquisitions and are ideal for single-cell imaging or imaging of (semi-) transparent embryos [19] . Unfortunately, they are not well suited for opaque mouse organs owing to poor sensitivity and high bleaching rate as well as limited penetration depth. More importantly, without any reproducibility in the heart's motion (as achieved with our stabilizer), these techniques can at best offer single-shot images rather than a complete imaging sequence over several cardiac cycles preventing signal averaging and dynamic imaging of the same physical plane within the heart. Indeed, cardiac motion is subject to 6 degrees of freedom in space, not only along the z direction. Even acquisition of hundreds or thousands of fast-shot images would likely not allow reconstructions of a single complete cardiac frame over time because of these misalignments. The above described system had a measured gated spatial resolution of 2×7 μm ( x / y versus z axis) using calibration beads lodged inside tissue. The ultimately achievable resolution, however, is primarily determined by the holder design and ring size. Future designs could be envisioned that further improve the resolution or coverage, for example, by changing the size or shape of the stabilizer or by increasing its contact area. Finally, similar holders and designs could be adapted to image other organs or orthotopic cancers at high resolution. Fabrication of stabilizer The custom-designed stabilizer was fabricated out of stainless steel with the overall dimensions shown in Fig. 1b and Supplementary Fig. S2 by using a standard benchtop milling machine. The outer diameter of the ring measured 3.6 mm, the inner diameter measured 2.2 mm and the height was 500 μm; the ring thus enabled imaging of a relatively large area. A shallow groove was carved out in the bottom of the ring to increase the contact area between the stabilizer and the bonding glue, and thus ensure better attachment to the heart. The stabilizer was fixed to a monolithic tristage base plate, which guarantees 6 degrees of freedom and allows small last-minute adjustments (displacements and/or rotations) to be made accurately and easily. Microscope An Olympus FV1000-MPE laser scanning microscopy system based on an upright BX61-WI microscope was used in either confocal or multiphoton mode. A tunable MaiTai DeepSee Ti:sapphire laser was used for two-photon microscopy. Two air objectives (XL Fluor 2×/340 NA 0.14; UPlanFL N 10× NA 0.30, Olympus) and a water-immersion objective with a high numerical aperture (NA) and large working distance (XLPlan N 25×, NA 1.05, working distance 2 mm, Olympus) were utilized. In addition, two miniaturized high-performance objectives (Stick Lenses) were used (6× IV-OB13F67W20, 20× IV-OB13F20W20; Olympus). Both objectives had a small diameter (1.3 mm) and a working distance of 200 mm. A custom-built Faraday cage was used to remove electromagnetic noise during ECG recordings. Mice A total of 40 mice were used for the experiments and their use was approved by the Institutional Review Board. Mice were anesthetized with 2% isoflurane and 2 l min −1 oxygen. The body temperature of the mice was kept constant at 37 °C during all procedures. Mice were placed on a surgical table in a supine position, and the trachea was intubated and ventilated using an animal ventilator (Harvard Apparatus INSPIRA ASV 55-7058). A thoracotomy was performed in the fourth left intercostal space. The heart was then exposed, all surrounding connective tissue was removed and the chest wall was kept open using a mini-retractor. Mice were moved to the microscopy stage on a heated glass plate (Olympus) to maintain body temperature. ECG traces were recorded via three subcutaneously placed needle electrodes in the forelimb and hindlimbs. The ECG signals were then amplified and filtered using a differential pre-amplifier (ADInstruments DP-301). The stabilizer ring was bonded to the epicardium using Dermabond (Ethicon). After imaging was complete, the thoracotomy was sutured with 5-0 nylon sutures (Ethicon) and the skin was sealed with additional Dermabond. Isoflurane was shut off and mice were extubated. Mice were then kept under observation for at least an hour with 100% oxygen flowing into the cage. Postprocedural analgesics (Buprenorphine) were given to all animals. Once the left ventricle could be visualized in vivo (described above), the imaging technique was applied to an ischaemia reperfusion model in mice. Ischaemia was induced by ligating the left coronary artery with an 8-0 monofilament nylon suture (Ethicon). After 30 min of ischaemia, the suture was removed to allow for reperfusion and each mouse was then either imaged or sewn back up, as described above. GFP cells were obtained from the bone marrow of ubiquitin–GFP mice. In these donor mice, the femur was excised and flushed, and the cells triturated through a nylon mesh filter (BD Bioscience) using a 3-ml syringe plunger. The cell suspension was subsequently centrifuged and the supernatant discarded. The cell pellet was resuspended in phosphate-buffered saline and kept on ice. The heart was visualized, as previously described. Fifty microlitre of the cell suspension was then injected into the left ventricular wall of the heart. Surgery was performed (as described above) 24 h before imaging. Cells were administered by apical intracardiac injection (away from the imaging site) to model stem cell engraftment procedures or given systemically to model circulating leucocyte biology. Imaging probes Rhodamine-labelled Griffonia simplicifolia lectin (RL-1102, Vector Laboratories) was used as an intravital stain to outline the microvasculature. The dose of the lectin was 50 μl of a 2 mg ml −1 solution, injected via a tail vein. The dye-labelled lectin, which has a maximum excitation at 550 nm and emission at 575 nm, was excited using a 559-nm laser. For multiphoton microscopy, the lectin was excited at 785 nm. Images were acquired at a speed of 15 frames per second using an optical zoom of X6 for all cell tracking experiments. Angiosense-680-IVM (NEV10065, Perkin Elmer) was used as a blood pool agent to observe functional vasculature. The dose of Angiosense was 150 μl at a dye concentration of 2 mol per mouse injected via tail vein. The agent, which has a maximum excitation at 680 nm and emission at 700 nm, was excited using a 635-nm laser. Rhodamine 6G dye (R4127, Sigma Aldrich) was used to stain leucocytes intravitally following intravenous injection [20] . One milligram of dye was dissolved in 1 ml of saline and injected at a concentration of 0.2 mg kg −1 via tail vein. The dye, which has a maximum excitation at 520 nm and emission at 550 nm, was excited using a 488-nm laser. Myocyte nuclei were labelled with Hoechst 33258 by applying it topically to the myocardium before imaging (50 μl of a 1/10,000 solution of Hoechst 33258). The dye, which has a maximum excitation at 352 nm and emission at 461 nm, was excited using a 352-nm laser. Data processing Data processing was done in real time, and all timing and pressure diagrams were recorded using a data acquisition card (DAQ, National Instruments). One PC (slave) was used to control the microscope electronics and acquire the images, while a second PC (master) was used to acquire all timing and physiological data ( Fig. 1a ). The master PC was connected to the slave PC via an Ethernet crossover cable to provide fast data transfer. Data were processed on a graphic processing unit for fast denoising ( Supplementary Figs S13 and S14 ) using a BM3D filter method [21] , [22] ; the data were likewise processed for real-time ECG parameter extraction using a well-established approach [23] , [24] , [25] . The latter determines the position of the QRS complexes and the beginning of the P waves. These analyses were critical for identifying the gating time window with minimal cardiac motion. All programming for data acquisition, data elaboration, noise reduction, ECG analysis and cell segmentation was done in Labview, Matlab, C++ and using the Cuda Toolkit. With the setup, we were able to choose either fast or slow image acquisition modes. Histology Following euthanasia and saline perfusion, hearts were embedded in optical cutting compound (Sakura Finetek), frozen in chilled isopentane and sectioned into 6-μm-thick slices. Sections were stained with anti-mouse CD11b antibody (clone: M1/70, BD Biosciences), a surface marker for myeloid cells, followed by biotinylated anti-rat IgG (Vector Laboratories Inc.). Avidin–biotin complex method was employed and the colour was developed by AEC substrate (Dakocytomation). MR imaging magnetic resonance imaging experiments were performed on a 7 Tesla Pharmascan (Bruker) system equipped with a mouse cardiac coil in birdcage design (Rapid Biomedical) to obtain cine volumetric short-axis images. Animals were anesthetized with 1% isoflurane by nose cone and placed into the coil in prone position. Electrodes were attached to the front left paw and right leg for ECG gating and monitoring of vital signs using a gradient echo sequence (echo time 2.6 ms, 16 frames per RR interval; flip angle 30°; in-plane resolution 200×200 μm; slice thickness 1 mm). The animals were kept warm by blowing hot air into the magnet. The air flow and the anaesthesia level were manually regulated to maintain the heart rate constant. How to cite this article: Lee, S. et al . Real-time in vivo imaging of the beating mouse heart at microscopic resolution. Nat. Commun. 3:1054 doi: 10.1038/ncomms2060 (2012).